Natural variation atXND1impacts root hydraulics and trade-off for stress responses inArabidopsis Soil water uptake by roots is a key component of plant performance and adaptation to adverse environments. Here, we use a genome-wide association analysis to identify the XYLEM NAC DOMAIN 1 (XND1) transcription factor as a negative regulator of Arabidopsis root hydraulic conductivity ( L p r ). The distinct functionalities of a series of natural XND1 variants and a single nucleotide polymorphism that determines XND1 translation efficiency demonstrate the significance of XND1 natural variation at species-wide level. Phenotyping of xnd1 mutants and natural XND1 variants show that XND1 modulates L p r through action on xylem formation and potential indirect effects on aquaporin function and that it diminishes drought stress tolerance. XND1 also mediates the inhibition of xylem formation by the bacterial elicitor flagellin and counteracts plant infection by the root pathogen Ralstonia solanacearum . Thus, genetic variation at XND1 , and xylem differentiation contribute to resolving the major trade-off between abiotic and biotic stress resistance in Arabidopsis . The growth performance and survival of terrestrial plants, whether in favorable or adverse environments, crucially depend on a proper uptake and management of water. Most plant species forage the soil for water through continuous growth and development of roots into a ramified architecture. The intrinsic water transport properties of root tissues (i.e., their root hydraulic conductivity, L p r ) are also important for efficient uptake and transfer of water towards the shoots. L p r shows a high environmental plasticity, with typical regulations depending on the availability of water, mineral nutrients or oxygen in the soil [1] . The same stimuli act on root growth and development, thereby altering root system architecture (RSA) [2] . Overall, growth and water transport properties of roots, which combine into the so-called root hydraulic architecture, determine the plant’s capacity to capture soil water under changing or heterogeneous soil conditions. Plants also display remarkable intraspecific genetic variations in RSA and hydraulics [3] , [4] , [5] , [6] , [7] , with possible impacts on abiotic stress responses. Thus, the ultimate question is to understand how combined genetic and physiological adjustments of RSA and root water permeability contribute to plant adaptation to specific habitats or climatic scenarios. Root water transport per se relies on several fundamental processes, often presented as sequential. Radial water flow, from the soil to the vasculature in the stele, is mediated through cell walls (apoplastic path) or from cell-to-cell. The latter path combines transcellular (across cell membranes and aquaporins) and symplastic (across plasmodesmata) transport. Water is then axially transported to the aerial parts through xylem vessels. The contexts in which root xylem can be hydraulically limiting are still debated [8] . Based on Poiseuille’s law of laminar flow, it was calculated that under water sufficient conditions this tissue is supposedly not limiting with respect to root structures mediating radial transport [9] . This may not be true in root tips, whereby vessels are not fully differentiated. Xylem cavitation under drought can also dramatically reduce plant hydraulic conductance and confer high plant vulnerability [10] . Conversely, drought impacts xylem differentiation further supporting a crucial role of vascular transport in these conditions [5] , [8] . However, this view may not apply to certain species or under mild water stress since intraspecific variation of xylem size in major crops such as rice was not associated to any growth advantage, especially under water deficit [11] . Thus, the links that xylem vessel differentiation establishes between root growth and development, hydraulics, and stress responses are not fully established [8] . In contrast, detailed studies have revealed how positioning of xylem axes contributes to early vascular pattern formation and how subsequent differentiation of xylem tracheary elements occurs through cell clearance by programmed cell death and deposition of lignin in secondary cell walls [12] . These developmental processes are controlled by regulatory networks involving NAC (NAM, ATAF1,2, and CUC2) [13] and MYB (myeloblastosis)-type transcription factors [14] . The former proteins have played a key evolutionary role in water-conducting structures from moss to vascular plants [15] . While root hydraulics is prone to fine biophysical analyses, genetic dissection of this trait has been somewhat lagging due in part to technical difficulties in defining proper hydraulic phenotypes. Reverse genetic analyses of candidate genes have uncovered the limiting role of aquaporins [1] or endodermal barriers [16] , [17] . In contrast, other components which determine root anatomy or environmental signaling and which can potentially interfere with root hydraulic properties have been poorly explored [18] . Quantitative genetics approaches based on intraspecific variations of root hydraulics [3] , [4] could help uncover such molecular components. In line with these ideas, quantitative trait locus (QTL) analysis of L p r in a biparental recombinant population (Bur-0 × Col-0) of Arabidopsis led to the cloning of hydraulic conductivity of root 1 , a Raf-like MAPKKK gene that acts as a negative regulator of L p r [19] . Here, we perform a genome-wide association analysis as another approach to identify genes controlling root hydraulics in Arabidopsis . We identify XYLEM NAC DOMAIN 1 ( XND1 ) as a key negative regulator of Arabidopsis root hydraulics at the species-wide level. Our study also reveals how genetic variation at XND1 may contribute to the trade-off between abiotic stress tolerance and biotic defense in Arabidopsis . A GWA study uncovers two novel genes controlling L p r A set of 143 Arabidopsis accessions from the RegMap panel [20] was phenotyped for root hydraulics (Supplementary Data 1 ). 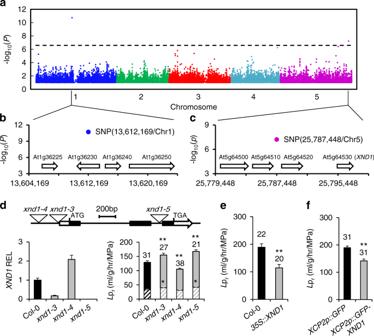Fig. 1 Identification ofXND1as a genetic determinant of root hydraulic conductivity.aManhattan plot of GWA for root hydraulic conductivity (Lpr) data based on a conditioned accelerated mixed-model. The chromosomes are depicted in different colors and thex-axis represents the chromosome number and position. A Bonferroni corrected significance threshold atα= 0.05 is indicated by the horizontal dashed line.b,cGene models of 20-kb genomic regions surrounding the two most significantly associated SNPs. The blue and purple dots represent these SNPs, and numbers onx-axes indicate chromosomal positions in base pairs.dMolecular and phenotypic characterization of threexnd1T-DNA insertion lines. The upper diagram shows a schematic representation of theXND1genomic region with positions of the three T-DNA insertions. The bar graph on the left showsXND1transcript abundance relative to Col-0 (relative expression level, REL) in thexnd1lines (means ± SE, based on two biological repeats). The bar graph on the right showsLprphenotypes before (whole bars) or after (hatched bars) root treatment for 30 min with the aquaporin blocker NaN3.e,fLprphenotype of Col-0 transgenic lines withXND1constructs under control of aCaMV35S(e) or a xylem specificXCP2Pro(XCP2p) (f) promoter. Inf, plants expressing GFP alone under the control ofXCP2Prowere used as negative controls. In all panels,Lprdata (means ± SE) were based on the indicated number of plants in two to three independent experiments. Asterisks indicate significant differences with respect to control lines (Student’sttest;*P< 0.05,**P< 0.01) A fourfold variation of L p r was observed among accessions (Supplementary Figure 1 ), with a coefficient of variation of 0.245 and a broad-sense heritability h 2 = 0.36. Conditional genome wide association (GWA) mapping using 250k single nucleotide polymorphisms (SNP) data [20] , and an accelerated mixed-model algorithm method with four markers as cofactors [21] revealed two SNPs that were significantly associated with L p r variation (Bonferroni multiple testing correction at α = 0.05) and contributed to 18.3% and 7.3% of the genetic variance, respectively (Fig. 1a ). One was located on chromosome (Chr) 1 (position 13,612,169), while the other was on Chr 5 (position 25,787,448). Considering 20-kb genomic regions surrounding these two association SNPs (Fig. 1b, c ), we identified eight candidate genes for L p r variation. 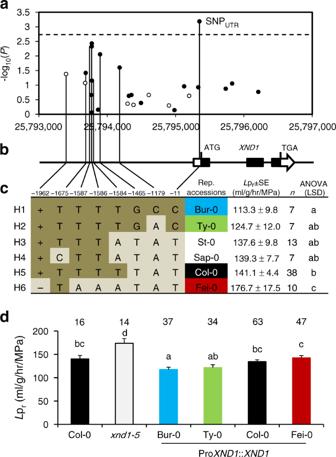Fig. 2 AXND1-based association analysis allows refining the natural allelic variations ofXND1.aThe association withLprof 27 polymorphic sites (MAF > 0.05) in the indicatedXND1genomic region was investigated in a set of 112 accessions. Thex-axis shows the nucleotide position of each variant, with empty and filled circles indicating INDELs and SNPs, respectively. They-axis shows the –log10(P) for the association tests, with the significance threshold atα= 0.05 indicated with a dashed line.bThe eight polymorphisms selected for further analysis are projected onto a schematic representation ofXND1gene structure. For position −1962, + and − represent an insertion and deletion, respectively. The boxes represent exons, with solid and empty boxes showing translated and untranslated regions, respectively. The SNP at Chr 5-P25,795,349 that surpassed the significance threshold inais located in the 5’-UTR ofXND1and indicated as SNPUTR.cThe eight selected nucleotide polymorphisms (with their distance from translation start site shown on the top) define six haplogroups (H1–H6). Representative accessions and meanLpr± SE within each haplogroup (n, accessions number) are shown. One-way ANOVA (Fisher’s LSD,P< 0.05) was used to test the significance of theLprdata.dTransgenic complementation ofxnd1–5with different allelic forms ofXND1. TheLprof Col-0,xnd1–5, andxnd1–5plants expressingXND1genomic fragments from Bur-0, Ty-0, Col-0, or Fei-0, was tested using 3–5 independent transgenic lines perXND1allele (see Supplementary Figure5). Mean values ± SE (n= 14–63 plants) are shown with sample size indicated on the top. One-way ANOVA (Fisher’s LSD,P< 0.05) was used to test the significance of the data None of these genes showed SNPs that were in strong linkage disequilibrium (LD) with the corresponding GWA studies (GWAS) peak SNP (Supplementary Figure 2 ). They were therefore further evaluated using a total of 15 Col-0-derived T-DNA insertion lines. As for the Chr1 region, two allelic insertion lines for At1g36240 showed, with respect to Col-0, an increase in L p r by 11 or 17%, while mutant lines for three neighboring genes did not show any significant L p r phenotype (Supplementary Table 1 ). When considering the four genes located in the Chr 5 region, we observed significantly altered L p r specifically for three T-DNA insertion lines of At5g64530 (Supplementary Table 1 ; Fig. 1d ). The data reveal the power of GWA mapping for identifying genetic determinants of specific traits like root hydraulics. At1g36240 encodes a putative ribosomal protein which will be investigated in another work. At5g64530 encodes Xylem NAC Domain 1 (XND1), a NAC transcription factors that antagonizes xylem differentiation, by negatively regulating secondary cell wall synthesis and programmed cell death [22] . Its putative function in axial water transport led us to examine in closer details its contribution to root hydraulics, which has not been described previously. Fig. 1 Identification of XND1 as a genetic determinant of root hydraulic conductivity. a Manhattan plot of GWA for root hydraulic conductivity ( L p r ) data based on a conditioned accelerated mixed-model. The chromosomes are depicted in different colors and the x -axis represents the chromosome number and position. A Bonferroni corrected significance threshold at α = 0.05 is indicated by the horizontal dashed line. b , c Gene models of 20-kb genomic regions surrounding the two most significantly associated SNPs. The blue and purple dots represent these SNPs, and numbers on x- axes indicate chromosomal positions in base pairs. d Molecular and phenotypic characterization of three xnd1 T-DNA insertion lines. The upper diagram shows a schematic representation of the XND1 genomic region with positions of the three T-DNA insertions. The bar graph on the left shows XND1 transcript abundance relative to Col-0 (relative expression level, REL) in the xnd1 lines (means ± SE, based on two biological repeats). The bar graph on the right shows L p r phenotypes before (whole bars) or after (hatched bars) root treatment for 30 min with the aquaporin blocker NaN 3 . e , f L p r phenotype of Col-0 transgenic lines with XND1 constructs under control of a CaMV35S ( e ) or a xylem specific XCP2Pro ( XCP2p ) ( f ) promoter. In f , plants expressing GFP alone under the control of XCP2Pro were used as negative controls. In all panels, L p r data (means ± SE) were based on the indicated number of plants in two to three independent experiments. Asterisks indicate significant differences with respect to control lines (Student’s t test; * P < 0.05, ** P < 0.01) Full size image XND1 negatively regulates root hydraulics Quantitative reverse transcription polymerase chain reaction (qRT-PCR) analyses revealed contrasting XND1 mRNA abundance in the three xnd1 allelic mutants (Fig. 1d ). xnd1–3 and xnd1–4 , which both exhibit a T-DNA insertion in the XND1 promoter region appeared as knock-down and activation lines, respectively. Consistent with a T-DNA insertion in the second intron, xnd1–5 can rather be considered as a knock-out allele. 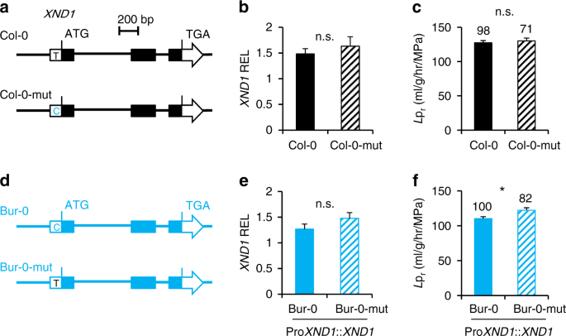Fig. 3 SNPUTRofXND1contributes toLprvariation. Transgenic complementation ofxnd1–5with Col-0 or Bur-0 allelic forms ofXND1, either wild-type or with a site-directed mutation at SNPUTR.a,dSchematic representation of investigatedXND1allelic forms. Col-0 and Bur-0 indicate the wild-type forms while Col-0-mut and Bur-0-mut indicate the corresponding point mutated forms.b,eTranscript abundance ofXND1inxnd1–5homozygous transgenic lines expressing the Col-0, Col-0-mut, Bur-0, or Bur-0-mut forms ofXND1. Three to five independent transgenic lines (two biological replicates for each) were studied for each form. Mean values ± SE (n= 18–30) were normalized to transcript abundance in Col-0.c,fLprof the transgenic lines described above. Three to five independent transgenic lines were phenotyped for each form. Mean values ± SE are shown with total number of plants indicated on the top. Student’sttest (*P< 0.05) was used to assess the statistical significance of the data (n.s. = not significant).XND1expression andLprdata in individual transgenic lines are shown in Supplementary Figure7 When considering the root dry weight (DW), primary and total root length, or lateral root density in plants grown in hydroponics, all three xnd1 genotypes had a root architecture similar to that of Col-0 (Supplementary Figure 3 ). In contrast, and by reference to Col-0, L p r was increased in hypofunctional mutants ( xnd1–3 , xnd1–5 ) by up to 29.7 ± 7.6% and decreased by 18.6 ± 4.7% in the xnd1–4 overexpression mutant. These results indicate that XND1 acts as a true negative regulator of root hydraulics. 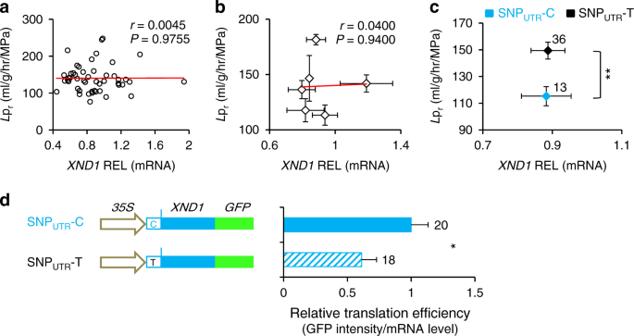Fig. 4 XND1-dependent natural variation ofLpris contributed by effects of SNPUTRon XND1 translation.a–cXND1transcript abundance was measured in the roots of 49 accessions using 6–10 plants and two independent experiments per accession. Data were analyzed considering each individual accession (a) or their grouping in the H1-H6 (b) or SNPUTR-C vs. SNPUTR-T haplogroups (c). Pearson correlation coefficient (r) andPvalue (P) betweenXND1transcript level andLprare shown inaandb. Error bars inbandcindicate SE. Accession number per haplogroup wasn= 3–18 inband as indicated inc(**P< 0.01 in Student’sttest).dA XND1–GFP fusion construct was placed downstream of aCaMV35Spromoter and aXND15’-UTR, with either C or T at SNPUTR. Note that this SNP is the only variation between Bur-0 and Col-0XND1alleles present in the construct sequence. Transcript abundance and fluorescence intensity of XND1–GFP was quantified in the roots of 9–10 transgenic lines per genotype, with two biological replicates. Relative translation efficiency of XND1–GFP was calculated in each individual line from the ratio of fluorescence to mRNA abundance. Mean values ± SE based on total number of lines and repeats are indicated on the right and were normalized to the data for SNPUTR-C. Student’sttest (*P< 0.05) was used to assess the statistical significance of the data Consistent with this, overexpression of XND1 under the control of a CaMV35S promoter (Supplementary Figure 4A, B ) resulted in a dramatic (−39.5 ± 7.7%) reduction in L p r (Fig. 1e ). XND1 is expressed in root xylem, preferentially in association with differentiating tracheary elements [22] , [23] . Transgenic expression of a GFP–XND1 fusion protein under the control of xylem specific promoter XCP2Pro (Supplementary Figure 4C , D ) reduced L p r by 25.3 ± 4.3% (Fig. 1f ), implying that XND1 acts in vascular tissues to exert hydraulic effects. Allelic diversity at XND1 validates GWA analyses The L p r associated SNP identified at position 25,787,448/Chr 5 during GWA analysis is located 7.9 kb apart from the XND1 coding region, whereas SNPs that are closer did not show any significant association. This hints to possible allelic heterogeneity and multiple mutations in XND1 that would contribute to L p r variation and are linked to the associated SNP. Newly released genomic sequences [24] were used to evaluate in closer details natural variation at XND1 among 112 accessions, of which 85 belong to the initially investigated panel while the remaining corresponds to accessions for which phenotypic data were generated later (Supplementary Data 2 ). Considering a genomic region from 2 kb upstream to 0.3 kb downstream of the XND1 coding region, we used a generalized linear model to test the association with L p r at 27 polymorphic sites (minor allele frequency (MAF) > 0.05), including SNPs and INDELs (Fig. 2a, b ). One single SNP located at position 25,795,349 in the 5′-UTR of XND1 surpassed the significance threshold and was thereafter named SNP UTR . Several SNPs also pointed to possible associations in the promoter region, consistent with putative allelic heterogeneity. Further, we used the eight polymorphisms showing the lowest P values ( P < 0.075) in this association analysis to define six haplogroups, each containing 7–38 accessions (Fig. 2c ; Supplementary Data 2 ). These haplogroups fall into four phenotypic classes with significant differences in mean L p r values (ANOVA; P < 0.05) (Fig. 2c ) suggesting that genetic diversity at XND1 truly contributes to shaping L p r variation at the species level. To establish this point further, we selected four accessions (Bur-0, Ty-0, Col-0, and Fei-0) as representative members of haplogroups with contrasting mean L p r values (Fig. 2c ). Corresponding genomic fragments encompassing XND1 were introduced into xnd1–5 and tested for their capacity to complement the mutant L p r phenotype (Fig. 2d ). 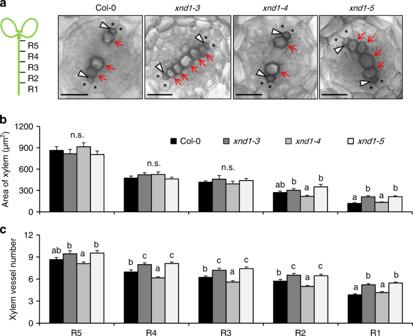Fig. 5 XND1 negatively regulates root xylem formation.aThe figure shows schematic representation of 2-cm-long segments (R1–R5) used for characterization of xylem anatomy in the indicated genotypes and representative cross-sections within the R2 segment. Arrowheads and arrows indicate protoxylem and metaxylem, respectively. Asterisks indicate pericycle cells adjacent to xylem poles. Scale bars represent 20 µm.b,cXylem area (b) and vessel number (c) (mean values ± SE) were measured in the indicated root segment and genotype, in 20–61 sections from 10–15 plants and 2–3 independent experiments. One-way ANOVA (Fisher’s LSD,P< 0.05) was used to test the significance of the data (n.s. = not significant) In these experiments, we used a set of three to five independent transgenic lines per haplotype, which provide mean XND1 expression levels similar to that in native Col-0 (Supplementary Figure 5A, B ). All four complemented series exhibited lower L p r than xnd1–5 , indicating that each of XND1 allelic forms was functional in a Col-0 background (Fig. 2d ; Supplementary Figure 5C ; Supplementary Data 3 ). In addition, transformation with the Bur-0 or Ty-0 alleles yielded lower L p r values than when using the Col-0 or Fei-0 allele, or the Fei-0 allele, respectively. Thus, with respect to Col-0 and Fei-0, the first two accessions harbor somewhat hyperfunctional alleles. Fig. 2 A XND1 -based association analysis allows refining the natural allelic variations of XND1 . a The association with L p r of 27 polymorphic sites (MAF > 0.05) in the indicated XND1 genomic region was investigated in a set of 112 accessions. The x -axis shows the nucleotide position of each variant, with empty and filled circles indicating INDELs and SNPs, respectively. The y -axis shows the –log 10 ( P ) for the association tests, with the significance threshold at α = 0.05 indicated with a dashed line. b The eight polymorphisms selected for further analysis are projected onto a schematic representation of XND1 gene structure. For position −1962, + and − represent an insertion and deletion, respectively. The boxes represent exons, with solid and empty boxes showing translated and untranslated regions, respectively. The SNP at Chr 5-P25,795,349 that surpassed the significance threshold in a is located in the 5’-UTR of XND1 and indicated as SNP UTR . c The eight selected nucleotide polymorphisms (with their distance from translation start site shown on the top) define six haplogroups (H1–H6). Representative accessions and mean L p r ± SE within each haplogroup ( n , accessions number) are shown. One-way ANOVA (Fisher’s LSD, P < 0.05) was used to test the significance of the L p r data. d Transgenic complementation of xnd1–5 with different allelic forms of XND1 . The L p r of Col-0, xnd1–5 , and xnd1–5 plants expressing XND1 genomic fragments from Bur-0, Ty-0, Col-0, or Fei-0, was tested using 3–5 independent transgenic lines per XND1 allele (see Supplementary Figure 5 ). Mean values ± SE ( n = 14–63 plants) are shown with sample size indicated on the top. One-way ANOVA (Fisher’s LSD, P < 0.05) was used to test the significance of the data Full size image To further investigate the significance of variation at XND1 , we revisited previous phenotyping data from a Bur-0 × Col-0 cross [19] . 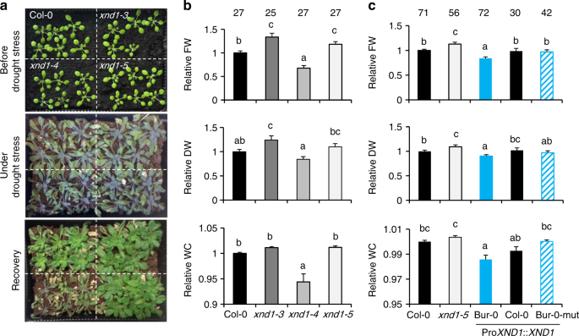Fig. 6 XND1 negatively regulates plant drought stress tolerance.aShoot phenotypes of Col-0 andxnd1plants at 22 days postgermination (upper panel), after water deprivation for 24 additional days (middle panel), and at 5 days after rewatering (lower panel).bRelative fresh weight (FW), dry weight (DW) and water content (WC) in shoots of indicated genotypes at 5 days after rewatering (seea). All data were normalized to values measured in Col-0 plants from the same pot. The figure shows mean values ± SE from the indicated number of plants and four biological replicates. One-way ANOVA (Fisher’s LSD,P< 0.05) was used to test the significance of the data.cSame parameters as inbbut for Col-0,xnd1–5, andxnd1–5plants complemented with the Bur-0, Col-0, or Bur-0-mutXND1alleles. Three to five independent transgenic lines were phenotyped for each allele. Mean values ± SE from the indicated number of plants are shown. One-way ANOVA (Fisher’s LSD,P< 0.05) was used to test the significance of the data Although there was no sign of a purely additive QTL at the bottom of Chr 5 in this cross [19] , we detected an epistatic QTL controlling L p r variation (Supplementary Figure 6 ), possibly including XND1 effect. The phenotypic consequence of segregation at XND1 region is conditioned by the allele present at a locus on Chr 2, suggesting that phenotypic expression of XND1 variation may depend on the genetic background. We note that, consistent with the effects of introducing a Bur-0 XND1 allele in Col-0 (Fig. 2d ), the RILs fixed for Bur-0 at XND1 region and Col-0 at the Chr2 locus exhibited a reduced L p r (Supplementary Figure 6 ). The overall genetic data validate the identification of XND1 by GWA mapping, and support the idea that allelic differences at XND1 contribute to the natural variation of L p r in Arabidopsis . A SNP in XND1 can account for natural variation of L p r Among the 112 accessions analyzed above, the SNP UTR , with C vs. T variation, identifies two haplogroups with significantly different L p r (SNP UTR -C, L p r = 114.8 ± 7.6, n = 16; SNP UTR -T, L p r = 145.5 ± 3.3, n = 96; P < 0.01). Bur-0 and Col-0 belong to the first and second haplogroups, respectively (Fig. 2c ). We addressed the functional significance of SNP UTR by transgenic complementation of xnd1–5 mutant with Bur-0 or Col-0 allelic forms of XND1 , either native or with a converting point mutation at SNP UTR (Fig. 3a, d ). While mutation of the Col-0 allele did not influence L p r (Fig. 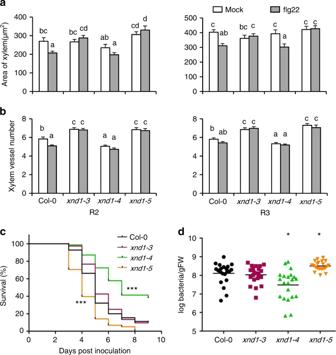Fig. 7 XND1 mediates the inhibition of xylem formation by flg22 and resistance toR. solanacearum.a,bPlants of the indicated genotype were grown for 4 days in the absence (mock) or in the presence of 0.25 µM flg22 (flg22). R2 and R3 root segments (see Fig.5a) were cross-sectioned and xylem area (a) and xylem vessel number (b) were measured. Data are means ± SE from 18–50 sections in 6–10 plants and two independent experiments. One-way ANOVA (Fisher’s LSD,P< 0.05) was used to test the significance of the data.cThe indicated genotypes were inoculated withR. solanacearumthrough root dipping and plant survival (in %) was scored at the indicated days postinoculation. Cumulated data from three independent biological experiments, each with three technical repeats comprising at least 24–32 plants. Stars indicate significant differences from Col-0 based on a Gehan–Breslow–Wilcoxon test (P< 0.0001). The Col-0 andxnd1–3curves were not significantly different (P= 0.1304).din plantagrowth measurement ofR. solanacearumat 3 days after inoculation of the indicated genotypes. Each dot represents a replicate of two plants and the black line indicates the mean of all the replicates. Cumulated data from four independent biological repeats. Asterisks indicate a significant difference with Col-0 (Mann–Whitney test; P< 0.05) 3b, c ; Supplementary Figure 7A, C ; Supplementary Data 4 ), the conversely mutated Bur-0 allele conferred a higher L p r than its native counterpart in xnd1–5 complemented lines (Fig. 3e, f ; Supplementary Figure 7B , D ; Supplementary Data 4 ). These data establish that SNP UTR contributes to natural variation of XND1 function. Since L p r phenotypic differences induced by these point mutations were in either case smaller than when comparing the two wild-type alleles (Fig. 2d ; Fig. 3c, f ), we hypothesize that other polymorphisms act, independently or in interaction with SNP UTR , to induce the full allelic effects. Effects of these polymorphisms would be more pronounced in the Col-0 allele than in the Bur-0 allele. Fig. 3 SNP UTR of XND1 contributes to L p r variation. Transgenic complementation of xnd1–5 with Col-0 or Bur-0 allelic forms of XND1 , either wild-type or with a site-directed mutation at SNP UTR . a , d Schematic representation of investigated XND1 allelic forms. Col-0 and Bur-0 indicate the wild-type forms while Col-0-mut and Bur-0-mut indicate the corresponding point mutated forms. b , e Transcript abundance of XND1 in xnd1–5 homozygous transgenic lines expressing the Col-0, Col-0-mut, Bur-0, or Bur-0-mut forms of XND1 . Three to five independent transgenic lines (two biological replicates for each) were studied for each form. Mean values ± SE ( n = 18–30) were normalized to transcript abundance in Col-0. c , f L p r of the transgenic lines described above. Three to five independent transgenic lines were phenotyped for each form. Mean values ± SE are shown with total number of plants indicated on the top. Student’s t test ( * P < 0.05) was used to assess the statistical significance of the data (n.s. = not significant). XND1 expression and L p r data in individual transgenic lines are shown in Supplementary Figure 7 Full size image Next, we addressed the general molecular mechanisms that can account for natural variation of XND1 function. Knowing that the XND1 allelic variation pointed by GWA and validated by transgenic complementation does not reside in the XND1 coding sequence, we investigated natural variation in XND1 expression and its potential functional significance. The abundance of XND1 transcripts was measured in the roots of 49 randomly selected accessions representative of the six previously defined H1–H6 haplogroups. No correlation of L p r with XND1 transcript abundance was observed when considering all individual accessions (Fig. 4a ), or their grouping in the H1–H6 (Fig. 4b ) or SNP UTR -C vs. SNP UTR -T (Fig. 4c ) haplogroups. Thus, the SNP UTR and other putative SNP(s) causing L p r variations have marginal effects, if any, on mRNA abundance at this scale. To investigate putative effects of SNP UTR on XND1 protein translation, a XND1-GFP fusion was placed under the control of a CaMV35S promoter and a XND1 5′-UTR, in its SNP UTR -C or SNP UTR -T form, and expressed in transgenic xnd1–5 (Supplementary Figure 8 ). Based on 9–10 lines per genotype with overall similar transcript abundance, we used GFP fluorescence as a reporter of XND1–GFP accumulation (Supplementary Figure 9A – D ). For each line, a relative translation efficiency was deduced from the ratio of XND1–GFP protein and mRNA abundances (Supplementary Figure 9E ). Combined data (Fig. 4d ) revealed that relative translation efficiency of the SNP UTR -C form was 63% higher than that of its SNP UTR -T counterpart. The positive effect of SNP UTR -C on XND1 translation and accumulation is consistent with lower L p r in the corresponding haplogroup. Fig. 4 XND1 -dependent natural variation of L p r is contributed by effects of SNP UTR on XND1 translation. a – c XND1 transcript abundance was measured in the roots of 49 accessions using 6–10 plants and two independent experiments per accession. Data were analyzed considering each individual accession ( a ) or their grouping in the H1-H6 ( b ) or SNP UTR -C vs. SNP UTR -T haplogroups ( c ). Pearson correlation coefficient ( r ) and P value ( P ) between XND1 transcript level and L p r are shown in a and b . Error bars in b and c indicate SE. Accession number per haplogroup was n = 3–18 in b and as indicated in c ( ** P < 0.01 in Student’s t test). d A XND1–GFP fusion construct was placed downstream of a CaMV35S promoter and a XND1 5’-UTR, with either C or T at SNP UTR . Note that this SNP is the only variation between Bur-0 and Col-0 XND1 alleles present in the construct sequence. Transcript abundance and fluorescence intensity of XND1–GFP was quantified in the roots of 9–10 transgenic lines per genotype, with two biological replicates. Relative translation efficiency of XND1–GFP was calculated in each individual line from the ratio of fluorescence to mRNA abundance. Mean values ± SE based on total number of lines and repeats are indicated on the right and were normalized to the data for SNP UTR -C. Student’s t test ( * P < 0.05) was used to assess the statistical significance of the data Full size image XND1 affects both xylem formation and aquaporin activity To understand further the causes of XND1 -mediated variation of L p r , we used sodium azide (NaN 3 ), a common blocker of plant plasma membrane aquaporins [3] , [19] . NaN 3 dramatically reduced L p r in Col-0 and three T-DNA insertion xnd1 genotypes, yielding a residual L p r , which was higher in loss-of-function alleles ( xnd1–3 , xnd1–5 ) than in wild type (Col-0) or gain-of-function ( xnd1–4 ) plants (Fig. 1d ). NaN 3 -resistant L p r accounts for aquaporin-independent water transport pathways, whether radial (apoplasm) or axial (xylem vessels). Here, facilitation of NaN 3 -resistant pathways in xnd1–3 and xnd1–5 is consistent with XND1 acting as a negative regulator of xylem differentiation. To assess this point, we probed xylem morphology along the root axis by sampling tissues in 2-cm-long consecutive segments from the root tip (Fig. 5 ). By comparison to Col-0, formation of the xylem (especially metaxylem) was advanced in xnd1–3 and xnd1–5 , while delayed in xnd1–4 (Fig. 5a ). Specifically, overall xylem area was enhanced in xnd1–3 and xnd1–5 in the most apical segment (R1) (Fig. 5b ). Xylem vessel number was consistently increased in several segments (R1–R4) of loss-of-function xnd1 alleles whereas it was reduced in the R2–R4 segments of xnd1–4 (Fig. 5c ). Fig. 5 XND1 negatively regulates root xylem formation. a The figure shows schematic representation of 2-cm-long segments (R1–R5) used for characterization of xylem anatomy in the indicated genotypes and representative cross-sections within the R2 segment. Arrowheads and arrows indicate protoxylem and metaxylem, respectively. Asterisks indicate pericycle cells adjacent to xylem poles. Scale bars represent 20 µm. b , c Xylem area ( b ) and vessel number ( c ) (mean values ± SE) were measured in the indicated root segment and genotype, in 20–61 sections from 10–15 plants and 2–3 independent experiments. One-way ANOVA (Fisher’s LSD, P < 0.05) was used to test the significance of the data (n.s. = not significant) Full size image We also observed that the absolute difference in L p r between Col-0 and xnd1 mutants was much higher in the absence than in the presence of NaN 3 (Fig. 1d ), suggesting that, with respect to Col-0, loss and gain-of-function xnd1 mutants show higher and lower plasma membrane aquaporin activity, respectively. Because XND1 serves as a transcription factor, we investigated whether it may alter, either directly or indirectly, the abundance of the corresponding aquaporin transcripts in roots. Thus, we considered all the 13 Plasma membrane Intrinsic Protein ( PIP ) genes and investigated the three T-DNA insertion xnd1 lines and XND1 overexpressors described above ( 35S::XND1 , XCP2p::GFP–XND1 ), taking Col-0 and XCP2p::GFP plants as controls. None of the PIP genes showed differences in expression that would correlate to L p r (Supplementary Figure 10 ), suggesting that effects of XND1 on aquaporin function are not mediated through PIP transcript abundance. The overall data indicate that XND1 acts as a negative regulator of L p r by repressing both xylem development and aquaporin activity. The latter effects are not yet understood and may well be indirect. XND1 negatively acts on plant drought stress tolerance By determining the efficiency of water supply to the plant’s aerial parts, root hydraulics can play a key role in maintaining the overall plant water status, especially in conditions of strong water demand or water deprivation. To investigate the general role of XND1 in plant water relations, we first compared the wild type (Col-0) and three xnd1 genotypes grown under various water regimes. Under sufficient water supply, all genotypes showed comparable growth performance, although xnd1–4 showed a slight deficit in shoot water content (Supplementary Figure 11A, B ). When seedlings were grown for three weeks in these favorable conditions and thereafter subjected to a long-term (24 days) water deprivation, all plant genotypes showed signs of severe stress and growth retardation, which, however, were the most pronounced in xnd1–4 (Fig. 6a ). Plant resilience to these extreme conditions was investigated at 5 days after rewatering. With respect to Col-0 plants, loss-of-function xnd1 mutants showed a higher shoot fresh weight (FW) and a tendency to higher shoot DW (Fig. 6b and Supplementary Figure 11C ). The gain-of-function xnd1 plants ( xnd1–4 ) showed a mirror phenotype with reduced shoot growth (lower FW and DW) and reduced shoot water content (Fig. 6b and Supplementary Figure 11C ). The overall data indicate that XND1 negatively acts on plant tolerance to water deficit. To address the significance of XND1 natural variation in plant drought tolerance, we investigated xnd1–5 lines complemented with the Bur-0, Col-0, or Bur-0 SNP UTR -mutated allelic forms of XND1 . Under water sufficient condition, all complemented lines showed comparable growth performance with respect to Col-0 and xnd1-5 , with a slight reduction in shoot water content in the Bur-0 allele complemented lines (Supplementary Figure 12 ). After successive drought and recovery, all complemented lines showed lower shoot FW than xnd1-5 indicating the functionality of the three XND1 allelic forms in these conditions (Fig. 6c and Supplementary Figure 13 ). Interestingly, complementation with the Bur-0 allele resulted in lower shoot FW than with the Col-0 or Bur-0 SNP UTR -mutated allele (Fig. 6c and Supplementary Figure 13 ). In addition, the shoot DW and water content of the Bur-0 allele complemented lines was lower than in lines containing the Col-0 or Bur-0 SNP UTR -mutated allele, respectively (Fig. 6c and Supplementary Figure 13 ). These differences establish that natural variation at XND1 , at the SNP UTR in particular, confers variations in integrated plant responses to drought. Fig. 6 XND1 negatively regulates plant drought stress tolerance. a Shoot phenotypes of Col-0 and xnd1 plants at 22 days postgermination (upper panel), after water deprivation for 24 additional days (middle panel), and at 5 days after rewatering (lower panel). b Relative fresh weight (FW), dry weight (DW) and water content (WC) in shoots of indicated genotypes at 5 days after rewatering (see a ). All data were normalized to values measured in Col-0 plants from the same pot. The figure shows mean values ± SE from the indicated number of plants and four biological replicates. One-way ANOVA (Fisher’s LSD, P < 0.05) was used to test the significance of the data. c Same parameters as in b but for Col-0, xnd1–5 , and xnd1–5 plants complemented with the Bur-0, Col-0, or Bur-0-mut XND1 alleles. Three to five independent transgenic lines were phenotyped for each allele. Mean values ± SE from the indicated number of plants are shown. One-way ANOVA (Fisher’s LSD, P < 0.05) was used to test the significance of the data Full size image XND1 contributes to protection against a vascular pathogen Plant vasculature serves as an infection route for pathogens and its development is targeted by multiple biotic factors. Along these lines, abundance of XND1 transcripts in Arabidopsis is enhanced up to fivefold by bacterial infiltration (e.g., Pseudomonas syringae pv. phaseolicola) and exposure to pathogen-associated molecular patterns (e.g., flg22) (see Arabidopsis eFP Browser database at http://bar.utoronto.ca/efp_arabidopsis/cgi-bin/efpWeb.cgi ). These data led us to examine in closer details the effects of flg22 on xylem formation. A treatment with 0.25 µM flg22 for 4 days reduced the overall xylem area in R2 and R3 segments of Col-0, but not in xnd1–3 or xnd1–5 (Fig. 7a ). In R2 root segments of Col-0, xylem vessel number was reduced by flg22 whereas it was unresponsive to the peptide in corresponding root segments of the three xnd1 insertion mutants (Fig. 7b ). Thus, XND1 mediates in part adjustments of vasculature formation under biotic constraints. The significance of these effects was further tested by exposing roots of various xnd1 genotypes to a soil borne pathogenic bacterium ( Ralstonia solanacearum) and scoring plant infection symptoms for up to 9 days (Fig. 7c , Supplementary Figure 14A ). Based on plant survival rate, the xnd1–3 knock-down line was indistinguishable from Col-0. In contrast, xnd1–5 and xnd1–4 showed, with respect to Col-0, a higher and lower susceptibility to the bacterial strain, respectively. Measurements of bacterial growth in rosettes confirmed this ranking, indicating that at 3 days postinoculation, xnd1–5 and xnd1–4 showed in planta bacterial multiplication that was higher ( P = 0.007) and lower ( P = 0.004), respectively, than in Col-0 (Fig. 7d ). At a later stage (4 days postinoculation), all genotypes exhibited similar bacterial contents (Supplementary Figure 14B ). Transformation of xnd1–5 with the Bur-0, Col-0, or Bur-0 SNP UTR -mutated allelic forms of XND1 abolished the higher susceptibility of xnd1–5 to R . solanacearum , with bacterial wilt phenotypes of the complemented lines similar to that of Col-0 (Supplementary Figure 14C ). The overall data indicate that XND1 limits bacterial proliferation in the plant and subsequent bacterial wilt appearance, supporting the idea that reduced xylem formation contributes to plant protection against bacterial infection. Fig. 7 XND1 mediates the inhibition of xylem formation by flg22 and resistance to R. solanacearum . a , b Plants of the indicated genotype were grown for 4 days in the absence (mock) or in the presence of 0.25 µM flg22 (flg22). R2 and R3 root segments (see Fig. 5a ) were cross-sectioned and xylem area ( a ) and xylem vessel number ( b ) were measured. Data are means ± SE from 18–50 sections in 6–10 plants and two independent experiments. One-way ANOVA (Fisher’s LSD, P < 0.05) was used to test the significance of the data. c The indicated genotypes were inoculated with R. solanacearum through root dipping and plant survival (in %) was scored at the indicated days postinoculation. Cumulated data from three independent biological experiments, each with three technical repeats comprising at least 24–32 plants. Stars indicate significant differences from Col-0 based on a Gehan–Breslow–Wilcoxon test ( P < 0.0001). The Col-0 and xnd1–3 curves were not significantly different ( P = 0.1304). d in planta growth measurement of R. solanacearum at 3 days after inoculation of the indicated genotypes. Each dot represents a replicate of two plants and the black line indicates the mean of all the replicates. Cumulated data from four independent biological repeats. Asterisks indicate a significant difference with Col-0 (Mann–Whitney test ; P < 0.05) Full size image Recent work from our group [19] has shown that, although technically challenging and under strong environmental and developmental dependency, root hydraulics ( L p r ) is amenable to quantitative genetics analyses. With respect to the recombinant population mapping approach used in our previous work, GWA studies could be more straightforward for identifying candidate genes quantitatively acting on a trait of interest. In any case, it is described that these two approaches are certainly complementary to reveal the genetic architecture of a trait [25] . In the present study, a one shot phenotyping of 143 accessions allowed identification of two novel genes, At1g36240 and At5g64530 , which proved to act as negative regulators of L p r . While additional work is required to assess the role of At1g36240, several complementary lines of evidence indicate that At5g64530 ( XND1 ) corresponds to the gene spotted by the GWA signal on Chr 5. First, loss- and gain-of-function of XND1 in Col-0 insertion mutants resulted in opposite L p r phenotypes. Although very encouraging to confirm our candidate gene’s association [26] , this is not sufficient per se. Thus, we also showed that four natural XND1 allelic forms have distinct abilities to complement the enhanced L p r phenotype of xnd1–5 knock-out plants. Remarkably, the corresponding haplogroups, each containing 7–38 natural accessions, showed consistent quantitative differences in L p r further supporting the idea that an allelic series at XND1 significantly modulates root hydraulics at the species-wide level. Additionally, an epistatic L p r QTL corresponding to the XND1 region was mapped in a Bur-0 × Col-0 RIL population, with effects on L p r consistent with those of corresponding XND1 alleles. Because of confounding genetic relatedness or allelic heterogeneities, the statistics of GWAS detection can lead to complex patterns where causal polymorphisms in the gene of interest are away from and do not show LD with the most significantly associated SNPs [27] . The present work may typically represent such case since the Chr 5 GWAS peak SNP (SNP peak ) was not in strong LD with any single SNP of neighboring genes in a 48 kb region (Supplementary Figure 2 ). Yet, a gene-based association study with a different accession set and an extended polymorphism data, pointed to a SNP present in the 5′-UTR of XND1 (SNP UTR ) as two allelic forms, and located at a 7901 bp distance from the Chr 5 GWAS peak SNP. The fact that SNP UTR and SNP peak do not appear in strong LD ( r 2 = 0.23, Supplementary Figure 2 ), could be explained in part by a bias due to the relatively low minor allele frequency (14%) at SNP UTR . Again, we used transgenic complementation to assess the functional significance of this variation: the contribution of this SNP UTR to L p r was established by site-directed allelic conversion of a Bur-0 allele and functional expression in a Col-0 background. Thus, the hyperfunctionality of the Bur-0 vs. Col-0 allele is due in part to a T-to-C substitution at this position. The failure of a symmetrical mutation in the Col-0 allele to modify L p r indicates that SNP UTR functionally interacts with other intragenic components to yield the XND1 -dependent variation of L p r . In particular, SNPs in the 3’UTR were not considered and could contribute to natural phenotypic variation. In summary, the overall work provides a thorough dissection of natural variations at XND1 and demonstrates their contribution to root hydraulics. Causal polymorphisms can be located in coding regions, in regulatory non-coding regions (this work) or can correspond to genomic structural variations [28] . Their identification usually provides highly relevant insights into the function and regulation of the gene or gene product of interest. In the case of XND1, two protein interaction motifs present in the C-terminal domain are essential for its function as they allow binding to the general cell cycle and differentiation regulator RETINOBLASTOMA-RELATED [29] . Yet, these motifs were highly conserved in the accession panel of this study and seem not to underlie XND1 -based natural variation of L p r . Here, we found that L p r natural variation was not correlated to XND1 transcript abundance when natural accessions were assembled in functionally discriminating haplogroups (Fig. 4b, c ; Supplementary Figure 15 ). Knowing that the 5′-UTR of plant genes can harbor regulatory elements that affect RNA structure, RNA–protein interactions and/or ribosome recruitment [30] , [31] , we investigated whether allelic variation at SNP UTR interferes with XND1 translation efficiency. Because XND1 is a transcription factor that is lowly abundant and primarily confined to the nucleus of xylem cells, we monitored fluorescence of a XND1–GFP construct in a specific root tip region as it was the most suitable to proper quantification. Although a definitive analysis such as ribosome profiling remains to be done, our results based on ratio of protein and mRNA abundances in cells ectopically expressing XND1 suggest that SNP UTR potentially affects translational efficiency. As a result, we propose that variation at SNP UTR leads to distinct XND1 protein abundance, xylem differentiation and L p r . We also stress that, as indicated by the local association study, SNP UTR is likely not the only causal SNP, and other variants, for instance specific to haplotype H6 (Fig. 2c ), may also be functional. The identification of XND1 in our GWA study was strikingly in line with the notion that NAC transcription factors control water-conducting structures from primitive terrestrial plants to most recently evolved vascular plants [15] , [22] , [32] . Further, XND1 is an angiosperm-specific NAC that contributes to specific vessel differentiation features in these plants [29] . Consistent with earlier studies [22] , we validated that XND1 negatively acts on xylem differentiation and, based on Hagen–Poiseuille law [33] , we propose that its developmental function results in an axial hydraulic limitation in root tips. A genetic link between xylem function and root hydraulics has previously been pointed by Lefebvre et al. [18] , based on the dramatic drop in L p r displayed by esk1 loss-of-function mutants. With respect to the general collapse of xylem vessels and pleiotropic stress phenotypes shown by these mutants, xnd1 genotypes showed milder alterations of xylem tissues, specifically in roots tips. Thus, a slightly altered abundance and overall size of the xylem vessels seem to be sufficient to perturb L p r . A more precise analysis indicated, however, that XND1 may also act on aquaporin function to reduce L p r . This could be due to indirect effects on aquaporin expression and/or function due to locally altered vascular tissue differentiation. While these conclusions rely on analysis of xnd1 transgenic lines, the precise mechanisms that underlie effects of natural XND1 variants on L p r remain to be explored. Beyond root hydraulics, our study underscores a general role of xylem in plant response to environmental stresses. In particular, we showed that XND1 negatively acts on drought tolerance. Based on the phenotype of XND1 overexpressors, we propose that reduced xylem differentiation and water transport in root tips hampers water extraction in deep, newly colonized soil strata. A reduced leaf water content was also observed in well-watered conditions, suggesting a general hydraulic limitation in these plants. These findings contribute to a longstanding debate on the role of xylem in drought tolerance. Genetic selection programs in wheat and rice have targeted xylem morphology using root thickness as a proxy [7] , [34] . However, the significance of these variations with respect to drought adaptation has been controversial (discussed by Lynch et al. [5] ). In wheat, reduced xylem diameter was linked to better growth in dry environments whereas, in rice, genotypic variation in xylem vessel diameter was not linked to the plant’s capacity to regulate leaf water status under drought [11] . The genetic variants of XND1 investigated in the present work provide more precise insights into these questions, at least in the case of Arabidopsis . We also realize that, besides efficiency for conducting the transpiration stream, xylem anatomy contributes to cavitation resistance and thereby to tolerance to extreme drought events. However, this critical trait, which shows high phenotypic and genotypic plasticity in trees [35] , could not be addressed in our work since no natural cavitation has ever been described in Arabidopsis . Xylem differentiation is sensitive to many more environmental factors than water availability [36] , [37] . For instance, a link between PAMP-triggered immunity and xylem differentiation pathways involving plant glycogen synthase kinase 3 proteins is emerging [38] , [39] . In the present work, we investigated the significance of XND1 induction by flg22, and found this gene to mediate the inhibiting effects of the elicitor on vascular formation. A general role for XND1 in plant defense was further investigated using R. solanacearum a prototypal root vascular pathogen that causes bacterial wilt in many plant species [40] . As for drought assays, series of hypo- and hyperfunctional, artificial and natural alleles were used to address XND1 function. Consistent with its induction upon infection, enhanced expression of XND1 in xnd1–4 led to plants more tolerant to R. solanacearum than Col-0, whereas a loss-of-function mutation ( xnd1-5 ) caused a mirror phenotype that could be complemented using either Col-0 or Bur-0 alleles. Several modes of actions may explain the role of XND1 in the present pathosystem. In agreement with in planta bacterial growth measurements, we propose that restriction or delayed differentiation of the vasculature mediated by XND1 may antagonize microbe propagation, and/or the establishment of an aqueous living space for pathogens [41] , thereby contributing to plant defense. Alternatively, and as shown for other NACs [42] , XND1-mediated transcriptional reprogramming could enhance plant immunity. Because of their general role in differentiation of water-conducting tissues, NACs have played a central role during plant evolution, and contributed to their adaptation to aerial environments [15] . Our study shows that natural selection is still at work in higher plants, and refines the role of a crucial NAC member in diverse vascular functions. By negatively acting on the differentiation of xylem vessels in root tips, XND1 sensitizes the plant to extreme drought events while directly or indirectly providing a partial protection against systemic pathogen attack. Thus, XND1 mediates a trade-off between plant responses to biotic and abiotic stresses. While environmental stresses can occur independently, sequentially or in combination, this work exclusively reports on effects of individual stresses. Since the role of XND1 could conceivably be more complex when stresses occur in concert than when applied individually, additional dimensions of the role of this gene in plant stress responses remain to be explored. Nevertheless, our work indicates that natural variation at XND1 may contribute to the extensive geographic distribution of species such as Arabidopsis [43] . Interestingly, the minor allelic form (14% of the 112 accessions) carrying SNP UTR -C was associated with hyperfunctional alleles, lower L p r and lower drought tolerance. This indicates that the selective balance of drought over pathogen attacks may have been predominant to maintain SNP UTR -T as the major allele. While our study emphasizes the adaptive significance of XND1 variations in natural plant populations, it will also be crucial to investigate the genetic variation of this gene and of other NAC homologs in trees [32] and herbaceous crops, for applied purposes such as wood quality, productivity under drought conditions or disease control. Plant materials Seeds for natural accessions of Arabidopsis thaliana (Supplementary Data 1 ) or T-DNA insertion lines (Supplementary Table 1 ) were obtained from the Nottingham Arabidopsis Stock Centre (NASC) except for seeds of FLAG_153A06 which came from the Versailles Arabidopsis Stock Center. When required, T-DNA insertions were confirmed by PCR using primers listed in Supplementary Table 2 . XND1 overexpression lines under control of a CaMV35S or xylem specific XCP2 promoter [44] were as described previously [22] , [29] . Hydroponic growth conditions Seeds were surface sterilized and sown on petri plates (12 × 12 cm, Gosselin, BP124-04) with 0.5 × Murashige and Skoog (MS) solid medium [2.2 g L −1 MS (Sigma, M5519), 10 g L −1 sucrose (Euromedex, 200–301 B), 0.5 g L −1 MES (Euromedex, EU0033), and 0.7% agar (Sigma, A4675), pH 5.7 adjusted using KOH]. Following stratification for 2 days in the dark at 4 °C, plates were incubated vertically for 9 days in a growth chamber at 20 °C and 70% relative humidity, with cycles of 16 h of light (250 µmol photons m −2 s −1 ) and 8 h of night. Plants were then transferred in hydroponic culture under the same growth conditions. The hydroponic medium (0.75 mM MgSO 4 , 0.5 mM KH 2 PO 4 , 1.25 mM KNO 3 , 1.5 mM Ca(NO 3 ) 2 , 50 µM Fe-EDTA, 100 µM Na 2 SiO 3 , 50 µM H 3 BO 3 , 12 µM MnSO 4 , 1 µM ZnSO 4 , 0.7 µM CuSO 4 , 0.24 µM Na 2 MoO 4 ) was replaced weekly. Root hydraulic conductivity ( L p r ) measurements Measurements were performed essentially as described [3] on 21- to 23-day-old plants cultured in hydroponics. The intact root system of a freshly de-topped plant was inserted into a pressure chamber filled with hydroponic solution (pH 6.5 adjusted using KOH), and sealed with a silicon dental paste (PRESIDENT Light Body, Coltene, Switzerland). The root system was subjected to a pressure pretreatment at 350 kPa for 10 min to attain equilibration of sap flow exuded from the hypocotyl section, and to successive treatments at 320, 160, and 240 kPa, each for 2 min. High-accuracy flow meters (Bronkhorst, France) in combination with a LabVIEW-derived application were used to record the rate of pressure ( P )-induced sap flow ( J v ). DW r was determined after desiccation at 80 °C for at least 24 h. L p r (in ml g −1 h −1 MPa −1 ) was calculated as: L p r = J v /(DW r ∙ P ). In azide (NaN 3 ) inhibition experiments, J v was measured at continuous 320 kPa and its percentage inhibition was measured at 30 min following the addition of 1 mM NaN 3 . GWA, candidate-based association and haplotype analysis For GWA analysis, L p r was measured on 143 natural accessions, each with 6 individual plants randomized over a measuring period of four weeks (Supplementary Data 1 ). For the calculation of broad-sense heritability, average intra-accession variance was taken as the environmental variance, and data for all individuals were used for calculating phenotypic variance. A conditional GWA analysis was conducted on mean L p r values using the GWAPP web interface ( https://gwas.gmi.oeaw.ac.at/ ) and the accelerated mixed-model (AMM) algorithm method with cofactors [21] . Genotype data for 206,087 SNPs from 250k SNP chip [20] were used to carry out GWA analysis, and only SNPs with MAF > 0.05 (equivalent to a minor allele count (MAC) ≥ 8) were considered. For conditional analysis, four successive steps were performed following an initial calculation with AMM. At each step, one among the nine most highly associated SNPs identified in the previous calculation was arbitrarily selected as a cofactor. In practice, four SNPs (Chr1-P13,612,169; Chr 5-P25,787,448; Chr 5-P21,846,701, and Chr4-P17,518,747) were stepwise included as cofactors. To correct for multiple testing, a Bonferroni correction with a nominal significance threshold ( α ) of 0.05 was applied, corresponding to an uncorrected P value of 2.61 × 10 −7 . The proportion of genetic variance explained by SNP (13,612,169/Chr1) and SNP (25,787,448/Chr 5) was determined using coefficients of determination from simple linear regressions. For XND1 -based local association analysis, we extracted from Salk Arabidopsis 1001 Genomes database ( http://signal.salk.edu/atg1001/index.php ) genomic sequences of XND1 (encompassing a region from 2 kb upstream to 300 bp downstream of XND1 coding sequence) from 112 accessions. Of these, 85 belong to the initially investigated panel for GWA mapping (Supplementary Data 2 ). Association analysis between polymorphic sites (including INDELs and SNPs with MAF > 0.05) and L p r were performed with TASSEL version 5 using a generalized linear model [45] . The significance threshold was set at a P value of 0.05 per marker number. Haplotypes were classified based on eight polymorphic sites showing the lowest P values according to XND1 -based local association analysis. The haplogroups containing at least five accessions were used for further comparative analysis. Genetic complementation of xnd1 A 7088 bp genomic region harboring XND1 was amplified from Col-0, Bur-0, Ty-0, and Fei-0 genomic DNA using a iProof High-Fidelity PCR Kit (Bio-Rad) and cloned into a pGreen0179 vector [46] . A QuikChange Site-Directed Mutagenesis Kit (Agilent stratagene) was used to mutate the SNP UTR (Chr5_P25,795,349) of the cloned Col-0 or Bur-0 XND1 fragments. All primer sequences used are listed in Supplementary Table 2 . The constructs were confirmed by sequencing and transferred into xnd1–5 mutant plants using the floral dip method [47] . For each construct, three to five independent homozygous transgenic lines were selected in T3 generation on 30 mg L −1 hygromycin B (Sigma), checked for XND1 expression (see below) and phenotyped for L p r . Quantitative gene expression XND1 and PIP mRNA abundance was characterized in transgenic lines and/or natural accessions using qRT-PCR. Total RNA was extracted from Arabidopsis roots and reverse-transcribed using a SV Total RNA Isolation System (Promega) and M-MLV reverse transcriptase (Promega), respectively. PCR was performed on an optical 384-well plate with a LightCycler ® 480 system (Roche) using SYBR Green I Master (Roche) or SYBR Premix Ex Taq (TaKaRa), according to the manufacturer’s instructions. TIP41-like protein (At4g34270), PP2A3 (At1g13320), and SAND family protein (At2g28390) were selected as reference genes [48] , based on their expression stability among accessions evaluated using a NormFinder software [49] . All primer sequences used are listed in Supplementary Table 2 . Relative expression levels were determined using the 2 (−ΔΔC(T)) method [50] , and calibrated with respect to transcript abundance in the wild-type control, unless otherwise stated. Characterization of RSA Roots of hydroponically grown 22-day-old plants were harvested and preserved in 20% ethanol solution. The whole root systems were immersed in water and positioned on a square petri dish (24 cm × 24 cm), so as to avoid root overlapping, and then imaged using an Epson V850 Pro scanner at 600 dpi. Primary and total root lengths, and lateral root density were analyzed with an OPTIMAS software (version 6.1). The lateral root density was determined on the primary root, in a 12 cm region starting from the tip. Root DW was determined after desiccation at 80 °C for at least 24 h. Root histological analyses Roots of 21- to 23-day-old plants were cut in 2-cm-long segments starting from 0.3 cm of the tip. Root segments were embedded in 4% low-melting point agarose (Euromedex, 1670-B) and cross-sectioned (~100 μm thickness) using a Micro-Cut H1200 Vibratome (Bio-Rad) according to the manufacturer’s instruction. Xylem morphology was observed under a BH-2 Bright field Microscope (Olympus) and quantified using ImageJ. Xylem vessels were identified from their thickened cell wall. Xylem size and abundance were assessed from the area of all vessels and vessel number, respectively. For testing the effect of flg22 on xylem formation, 19-day-old plants were exposed for 4 days to a hydroponic solution containing 0.25 µM flg22 or 0.025% DMSO as mock treatment, and xylem morphology was analyzed as described above. Expression of fluorescent XND1 fusion proteins A 1465 bp region harboring XND1 5′-UTR and coding sequence, without stop codon and in its wild-type or SNP UTR -mutated Bur-0 form, was amplified from above mentioned XND1 -pGreen0179 clones. The fragment was cloned using the Gateway Technology (Invitrogen), downstream of a 35SCaMV promoter and in fusion with GFP in a pGWB505 vector [51] . The primers used are listed in Supplementary Table 2 . The constructs were confirmed by sequencing and transferred into xnd1–5 mutant plants. For each construct, nine to ten independent transgenic lines were selected in T2 generation on 30 mg L −1 hygromycin B (Sigma), cultured in hydoponics and checked for XND1-GFP transcript abundance and GFP fluorescence intensity in roots. The primers used for qRT-PCR are listed in Supplementary Table 2 . For quantification of the GFP fluorescence intensity, roots of 21- to 23-day-old plants were observed using a fluorescence microscope (Zeiss Axio Observer 7) and mean gray values in 400 µm root tips were quantified using an ImageJ program (NIH, USA). Data were normalized to the corresponding value of the line C9-3, which possessed the lowest transcript abundance and fluorescence intensity. Drought stress treatments Col-0 plants, xnd1 T-DNA insertion and complementation lines were grown in trays filled with peat soil (Neuhaus Humin Substrat N2, Klasmann-Deilmann). Four to six trays were used per experiment. Each tray was divided in four quarters, each containing six plants of a specific genotype (quarter-split manner). The dimensions (length × width × depth) of the trays were 18 cm × 13 cm × 5.5 cm. Plants were maintained in a growth chamber at 20 °C and 65% relative humidity, with cycles of 8 h of light (250 µmol photons m −2 s −1 ) and 16 h of night, and sufficient watering. After 22 days, plants were subjected to drought by withholding water for 24 days and re-irrigated for 5 days. Gravimetric soil water content was around 30% at the end of the water deficit period. The control treatment was conducted in the same conditions, but with continuous watering. Shoot fresh weight (FW) was determined immediately after harvest whereas shoot DW was measured after further desiccation for at least 4 days at 60 °C. Shoot water content was calculated as the FW-to-DW difference. All data were normalized to the corresponding mean value of Col-0 plants in the same tray. Bacterial inoculations Seeds of Col-0 plants and xnd1 T-DNA insertion lines were surface sterilized for 20 min with a 12% sodium hypochlorite solution, washed five times with sterile water and sown on a MS solid medium. After 8 days at 20 °C in a growth chamber, plantlets were transferred to Jiffy pots (Jiffy France, Lyon, France) and grown for 3 weeks under short days conditions at 22 °C and 70% relative humidity with 9 h of light (250 μmol m −2 s −1 ). Exposed roots of the plants were immersed for 20 min in a suspension containing 10 8 bacteria/mL of R. solanacearum GMI1000 strain [52] . Inoculated plants were then transferred to a new tray on a firm surface of potting soil, and incubated in a growth chamber at 75% relative humidity with cycles of 12 h of light (100 μmol m −2 s −1 ) at 27 °C and 12 h of night at 26 °C. Plant position was randomized prior to inoculation. Symptom appearance was scored daily and independently for each plant, using a macroscopic scale describing the observed wilting: 0, no wilting; 1, 25% of leaves wilted; 2, 50%; 3, 75%; 4, complete wilting. For subsequent analysis, the data were transformed into a binary index: 0, < 50% leaves wilted; 1, ≥ 50% wilted leaves in order to construct survival curves. We then applied the Kaplan–Meier survival analysis [53] with the Gehan–Breslow–Wilcoxon method to compute the P value and test the null hypothesis of identical survival experience of the tested mutant. A P value lower than 0.05 was considered to be significant. The survival curves represent a pool of three technical replicates, each with 24–32 plants, and 3 independent biological replicates corresponding to 240 plants for Col-0 and for each of the xnd1 T-DNA insertion lines. For bacterial internal growth measurements, a R. solanacearum GMI1000 derivative strain carrying a gentamycine resistance cassette [54] was used. Rosettes of three to six pairs of plants were harvested at 3 and 4 days postinoculation, sterilized in 70% ethanol and rinsed three times in sterile water. The rosettes were then weighted, grinded and re-suspended in sterile water. Bacterial concentrations were determined by plating dilutions on B medium. Four biological replicates were done. Comparison of in planta bacterial multiplication in xnd1 genotypes with that in Col-0 was performed through a Mann–Whitney test. All statistical analyses were performed with a Prism version 5.0 software (GraphPad Software, San Diego, CA, USA). Statistical analyses Unless otherwise indicated, statistical significance of the data was assessed using either a Student’s t test ( * P < 0.05) or one-way ANOVA (lowercase letters: P < 0.05). Student’s t tests were performed using EXCEL whereas a STATISTICA software was used for ANOVA and multiple comparison tests (Fisher’s least significant difference).